Mobile uranium(IV)-bearing colloids in a mining-impacted wetland Tetravalent uranium is commonly assumed to form insoluble species, resulting in the immobilization of uranium under reducing conditions. Here we present the first report of mobile U(IV)-bearing colloids in the environment, bringing into question this common assumption. We investigate the mobility of uranium in a mining-impacted wetland in France harbouring uranium concentrations of up to 14,000 p.p.m. As an apparent release of uranium into the stream passing through the wetland was observable, we examine soil and porewater composition as a function of depth to assess the geochemical conditions leading to this release. The analyses show the presence of U(IV) in soil as a non-crystalline species bound to amorphous Al-P-Fe-Si aggregates, and in porewater, as a distinct species associated with Fe and organic matter colloids. These results demonstrate the lability of U(IV) in these soils and its association with mobile porewater colloids that are ultimately released into surface water. Uranium, a radioactive element used in the weapon and nuclear energy industries, is a source of contamination at numerous sites around the world owing to its mining, milling and processing at large scales. Moreover, naturally occurring high U concentrations in ground and surface water are common in alpine regions [1] , [2] where the surrounding granitic bedrock contains trace amounts of uranium [3] . Wetlands often act as sinks for U and other trace metals and U has been shown to accumulate in wetland soils up to several thousand p.p.m. [1] , [2] . In natural settings, U occurs in the hexavalent [U(VI)] or tetravalent [U(IV)] oxidation states [4] . Because of the relatively high stability and low solubility of uraninite (U IV O 2 ) under reducing conditions at near-neutral pH, its formation as a result of (bio)reduction is considered an efficient strategy for U immobilization in sediments [5] . A similar reductive immobilization process is sought in constructed wetland systems [6] . Thus, U(IV)—where it occurs in the environment—is generally expected to be a low mobility U species, in contrast to U(VI) species that are generally soluble and mobile. Recently, non-crystalline U(IV) species were discovered as the product of microbial U(VI) reduction in batch experiments [7] , [8] , flow-through columns with natural sediments [9] and in field biostimulation [10] . It was also demonstrated that non-crystalline U(IV) was formed by the reduction of dissolved U(VI) by vivianite (Fe 3 (PO 4 ) 2 ) or phosphate-sorbed magnetite (Fe 3 O 4 ) [11] . These non-crystalline species are being characterized in ongoing research but are commonly referred to as ‘monomeric U(IV)’ in reference to the lack of U–U pair correlations as observed in their X-ray absorption spectroscopy (XAS) spectra [7] . A wetland in central France located adjacent to a former U mine was affected by mining activity for several decades. A recent study showed that there were hotspots within the wetland with soil U concentrations of up to 4,000 p.p.m. [12] . Here we show that the U concentration in a stream flowing through the wetland increases as a function of distance, suggesting U release into the stream. Major elements and U speciation analysis in porewater and soil as a function of depth allows linking of U(IV) mobilization in the porewater to its association with Fe and organic matter (OM) colloids. Furthermore, U in the soil occurs primarily as monomeric U(IV), more specifically, a U(IV) species bound to amorphous Al-P-Fe-Si aggregates through phosphate groups. The results imply that the non-crystalline form of U(IV) extant in the soil is labile and may complex with mobile Fe and OM colloids that are ultimately released into the stream. The environmental implication of these findings is that, currently, U(IV) mobility may be severely underestimated in high OM environments such as wetlands. Study site The studied wetland is located in the Limousin region of France, in the northwestern part of Massif Central, where igneous rocks such as granite dominate. A former open-pit and underground U mining site with adjacent waste rock piles and a high U clay deposit are located north of the wetland, which represents the lowest topographical point ( Fig. 1 ). A stream flows through the wetland. Two locations harbouring high U concentrations, henceforth referred to as ‘spot A’ and ‘spot B’, were identified in the site after a gamma radiation survey. Spot A is located south of the eastern waste rock pile and the high U clay deposit; spot B is adjacent to the western waste rock pile ( Fig. 1 ). 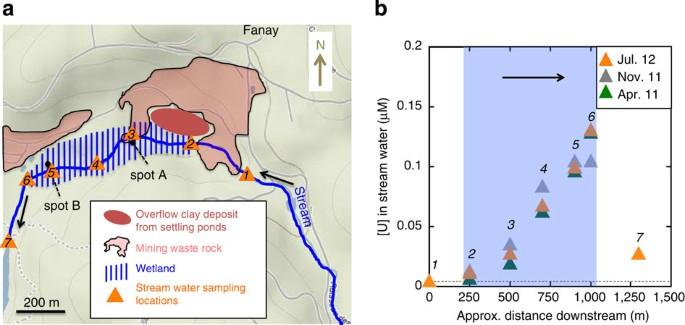Figure 1: Site map and U content in the stream. (a) The two black arrows show the stream flow direction and the seven numbered orange triangles indicate locations where stream water was sampled in April and November 2011 and July 2012 (locations number 1 and 7 outside the wetland were only sampled in July 2012). (b) U concentration data for the sampled stream water in the three seasons indicate a clear increase with distance downstream within the wetland and a decrease in the lake inlet because of dilution from lake water, which suggests that U is released gradually into the stream water from the wetland; the black arrow shows the stream flow direction; the blue zone shows the distance range within the wetland; the dashed line represents the background U concentration (0.0042 μM) for surface water in the region. The stream water samples were filtered with 0.22 μm pore-size membrane. The highest s.d. (Δ) is 10% of the reported values based on three replicate measurements and is not shown. Figure 1: Site map and U content in the stream. ( a ) The two black arrows show the stream flow direction and the seven numbered orange triangles indicate locations where stream water was sampled in April and November 2011 and July 2012 (locations number 1 and 7 outside the wetland were only sampled in July 2012). ( b ) U concentration data for the sampled stream water in the three seasons indicate a clear increase with distance downstream within the wetland and a decrease in the lake inlet because of dilution from lake water, which suggests that U is released gradually into the stream water from the wetland; the black arrow shows the stream flow direction; the blue zone shows the distance range within the wetland; the dashed line represents the background U concentration (0.0042 μM) for surface water in the region. The stream water samples were filtered with 0.22 μm pore-size membrane. The highest s.d. (Δ) is 10% of the reported values based on three replicate measurements and is not shown. Full size image Increase of U concentration in the stream Stream water was sampled at various locations in three seasons and analysed for U content ( Fig. 1 ). A steady increase of the stream concentration of soluble U from 0.012 to 0.13 μmol l −1 as a function of distance was observed, and this increase is proposed to correspond to the release of U into the stream. Hence, it was important to investigate the geochemical conditions leading to this release. Porewater chemistry Profiles of porewater dissolved oxygen (DO), SO 4 2− , Fe(II), Fe T and U ( Fig. 2 ) at spots A and B in November 2011 and July 2012 show a suboxic-anoxic environment where Fe(III) reduction—of possible microbial origin—as well as, to a lesser extent, sulphate reduction occur. At spots A and B, sulphate reduction proceeds as evidenced by the decreasing concentration of sulphate with depth and the presence of small concentrations of sulphide (1–4 μM) in the porewater ( Supplementary Fig. S1 ). This process is more prevalent at spot B than at spot A, as X-ray diffraction (XRD) analysis shows the presence of pyrite in the soil at spot B at 30–40 cm but not at spot A ( Supplementary Fig. S2 ). Sulphate reduction is unlikely to be a major process here because of the persistence of substantial porewater Fe(II) concentrations at both locations ( Fig. 2 ). Fe(III) reduction is clearly ongoing due to the presence of high concentrations (up to ~400 μM) of Fe(II), which represents the entirety of Fe in the porewater. Hence, reducing conditions prevail throughout the depth profile with some seasonal excursions of the redox front in the top 40 cm. Most interestingly, despite reducing conditions, U content in the porewater is significant with a spot A average U concentration of 0.80±0.20 μM in November and 0.91±0.07 μM in July and up to 3 μM at spot B in November. 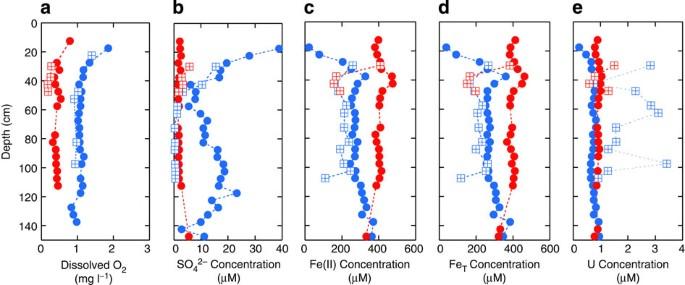Figure 2: Porewater chemistry. The profiles of (a) DO, (b) SO42−, (c) Fe(II), (d) FeTotaland (e) U in the porewater at spots A and B in November 2011 and July 2012. Blue circle: spot A November 2011; red circle: spot A July 2012; blue-crossed square: spot B November 2011; red-crossed square: spot B July 2012. The samples were filtered with 0.22 μm pore-size membrane. The porewater pH value is 5.8±0.2 in both seasons (Supplementary Fig. S1). The measured porewater temperature is 7–10 °C and 17–22 °C in November and July, respectively. Relatively fewer data points are available at spot B as compared with spot A because of the fact that numerous sampling chambers at spot B did not hold sufficient water to allow reliable porewater collection. The s.d. (Δ) is <5% of the reported values based on three replicate measurements and is not shown. Figure 2: Porewater chemistry. The profiles of ( a ) DO, ( b ) SO 4 2− , ( c ) Fe(II), ( d ) Fe Total and ( e ) U in the porewater at spots A and B in November 2011 and July 2012. Blue circle: spot A November 2011; red circle: spot A July 2012; blue-crossed square: spot B November 2011; red-crossed square: spot B July 2012. The samples were filtered with 0.22 μm pore-size membrane. The porewater pH value is 5.8±0.2 in both seasons ( Supplementary Fig. S1 ). The measured porewater temperature is 7–10 °C and 17–22 °C in November and July, respectively. Relatively fewer data points are available at spot B as compared with spot A because of the fact that numerous sampling chambers at spot B did not hold sufficient water to allow reliable porewater collection. The s.d. (Δ) is <5% of the reported values based on three replicate measurements and is not shown. Full size image The reducing conditions that persist in this soil support the hypothesis that U is present in a reduced tetravalent form. Metal- and sulphate-reducing bacteria have been shown to enzymatically and indirectly reduce U(VI) [13] , [14] . To elucidate the valence state of porewater U, laser-induced fluorescence spectroscopic (LFS) analysis was conducted on selected spot A porewater samples (November, 15–20 cm and 35–40 cm; and July, 15–20 cm) and on the same samples oxidized by atmospheric oxygen as positive controls. The results ( Supplementary Fig. S3 ) show a detectable U(VI) luminescence signal at ~493 and ~514 nm for the oxidized control samples. In contrast, the signal of the original samples was within the background noise. Thus, these results reveal that the predominant U redox state in porewater is tetravalent. The relatively high U(IV) porewater concentrations are surprising because in this valence state, U is sparingly soluble at the porewater pH value (5.8). Dissolved OM may complex and stabilize U(IV) in aqueous phases [15] , which is consistent with high dissolved organic carbon values in the porewater (1.24±0.06 mM, Supplementary Fig. S1 ). In addition, U may be bound to colloidal phase(s) smaller than the filter pore size (0.22 μm). Characterization of U-bound porewater colloids To probe the potential for the presence of colloidal U in the porewater, freshly collected samples maintained under anoxic conditions were subjected to immediate on-site ultrafiltration. Porewater from selected depths at spot A was divided into subsamples that were filtered through membranes with pore sizes of 0.22 μm, 500 or 10 kDa ( Fig. 3 ). At all depths investigated, 93–98% of U was present in the 500-kDa–0.22 μm size fraction along with >50% of Fe and 40–56% of organic carbon (OC). This finding supports the hypothesis that the high U concentration in the porewater is due to its association with Fe(II)-rich and OM-rich colloids. 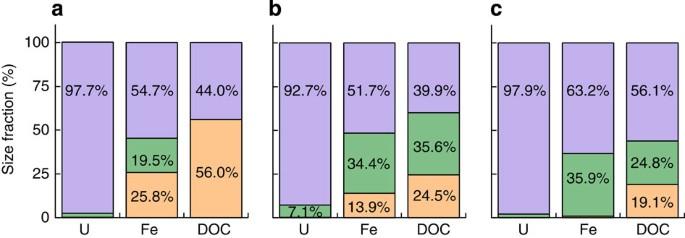Figure 3: Porewater ultrafiltration. The ultrafiltration results obtained from selected porewater samples from spot A collected in July 2012. Purple: 500 kDa–0.22 μm; green: 500 kDa–10 kDa; orange: <10 kDa. (a) For porewater at 15–25 cm depth, the total U, Fe and OC concentrations in the aqueous phase filtered with 0.22 μm pore-size membrane are 0.81 μM, 427 μM and 3.74 mM, respectively. (b) For porewater at 60–75 cm depth, the total U, Fe and OC concentrations in the aqueous phase filtered with 0.22 μm pore-size membrane are 0.90 μM, 402 μM and 2.61 mM, respectively. (c) For porewater at 115–130 cm depth, the total U, Fe and OC concentrations in the aqueous phase filtered with 0.22 μm pore-size membrane are 1.08, 423 and 2.35 mM, respectively. The s.d. (Δ) is <5% of the reported values based on three replicate measurements and is not shown. Figure 3: Porewater ultrafiltration. The ultrafiltration results obtained from selected porewater samples from spot A collected in July 2012. Purple: 500 kDa–0.22 μm; green: 500 kDa–10 kDa; orange: <10 kDa. ( a ) For porewater at 15–25 cm depth, the total U, Fe and OC concentrations in the aqueous phase filtered with 0.22 μm pore-size membrane are 0.81 μM, 427 μM and 3.74 mM, respectively. ( b ) For porewater at 60–75 cm depth, the total U, Fe and OC concentrations in the aqueous phase filtered with 0.22 μm pore-size membrane are 0.90 μM, 402 μM and 2.61 mM, respectively. ( c ) For porewater at 115–130 cm depth, the total U, Fe and OC concentrations in the aqueous phase filtered with 0.22 μm pore-size membrane are 1.08, 423 and 2.35 mM, respectively. The s.d. (Δ) is <5% of the reported values based on three replicate measurements and is not shown. Full size image Further characterization of U-bearing colloids using transmission electron microscopy (TEM) revealed a morphology reminiscent of beads on a string ( Fig. 4 and Supplementary Fig. S4 ). Elemental mapping shows that these colloids are composed of Fe and C, suggesting OM threads extending for hundreds of nanometres with associated iron-rich nanoparticles. Point energy-dispersive X-ray spectroscopy (EDS) analyses show low but statistically relevant U concentrations in association with Fe and C ( Supplementary Table S1 ). High-resolution transmission electron microscopic (HRTEM) observation reveals that string-associated crystalline nanoparticles of 2–3 nm and selected area electron diffraction (SAED) patterns are consistent with a mixture of trigonal Fe II (OH) 2 and cubic Fe II O nanoparticles ( Fig. 4 ). Fe II O probably resulted from the sintering of Fe(OH) 2 particles under the intense electron beam during SAED data collection. Altogether, these U-bearing colloids consist of Fe II (OH) 2 associated with OM as anisotropic threads that could pass through a 0.22-μm pore-size membrane but are retained by a 500-kDa pore-size filter. A previous study showed that OM-rich colloids with associated Fe and Ca precipitates were found in porewater of a wetland-karst system in Switzerland [16] , suggesting that this type of Fe- and OM-rich colloids may be common in mineral-rich wetland environments. 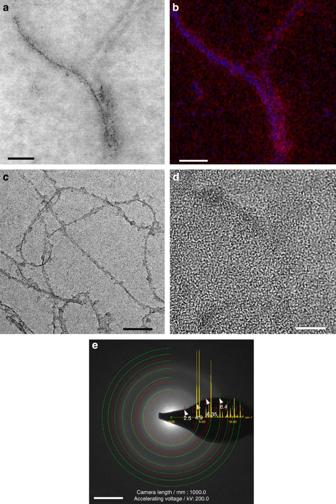Figure 4: TEM observation of U-containing colloids in porewater. (a) Scanning TEM image of colloids in porewater at 15–20 cm depth at spot A that was filtered with 0.22 μm pore-size membrane; (b) the corresponding Fe (blue)/C (red) EDS map; (c) TEM image of colloids in the same sample; (d) HRTEM image of small crystallites; (e) SAED pattern obtained from similar colloids interpreted as a combination of trigonal Fe(OH)2(red) and cubic FeO (green) phases. Point EDS analyses on similar colloids show low but statistically relevant U concentrations in association with Fe and C (Supplementary Table S1). Similar results obtained from other selected porewater samples are shown inSupplementary Fig. S4. Scale bar, 50 nm (a,b); 100 nm (c); 5 nm (d); 5 nm−1(e). Figure 4: TEM observation of U-containing colloids in porewater. ( a ) Scanning TEM image of colloids in porewater at 15–20 cm depth at spot A that was filtered with 0.22 μm pore-size membrane; ( b ) the corresponding Fe (blue)/C (red) EDS map; ( c ) TEM image of colloids in the same sample; ( d ) HRTEM image of small crystallites; ( e ) SAED pattern obtained from similar colloids interpreted as a combination of trigonal Fe(OH) 2 (red) and cubic FeO (green) phases. Point EDS analyses on similar colloids show low but statistically relevant U concentrations in association with Fe and C ( Supplementary Table S1 ). Similar results obtained from other selected porewater samples are shown in Supplementary Fig. S4 . Scale bar, 50 nm ( a , b ); 100 nm ( c ); 5 nm ( d ); 5 nm −1 ( e ). Full size image Characterization of stream colloids To elucidate the relationship between the steady increase in U concentration along the stream and the presence of mobile U-bearing colloids in the porewater, colloids in filtered stream water were analysed for their chemical composition and mineralogy. They were composed mainly of OC (26.6% w/w), Fe (22.3%), Si (1.9%), Ca (1.0%), Al (0.8%) and U (0.2%). Fe and OC, the main elemental components, are in an XRD amorphous phase(s) ( Supplementary Fig. S2 ). These stream colloids thus bear an uncanny compositional resemblance to the U-bearing porewater colloids (that is, they are rich in Fe and OC and contain U). Characterization of soil and U speciation Soil samples from both spots A and B are rich in water (65–90% w/w in most cases). Chemical composition profiles in the soil show a U- and Fe-rich layer at 0–30 cm and 0–40 cm at spots A and B, respectively ( Supplementary Fig. S5 ). Total organic carbon (TOC) content (w/w) in dried soil shows similar low average values at both spot A (16.3%±7.5%) and spot B (19.4%±7.4%), suggesting high mineral content. The Al and Si profiles, along with the XRD analysis ( Supplementary Fig. S2 ), underscore the presence of aluminosilicates in the soil. Images of the cores ( Supplementary Fig. S6 ) show the presence of a distinct clay-like layer at 10–25 cm for spot A and at 10–30 cm for spot B. XRD analysis confirmed the presence of muscovite (KAl 3 Si 3 O 10 (OH) 2 ), smectite ((Ca 0.5 ,Na) 0.7 (Al,Mg,Fe) 4 [(Si,Al) 8 O 20 ]·nH 2 O), albite (NaAlSi 3 O 8 ), orthoclase (KAlSi 3 O 8 ) and kaolinite (Al 2 Si 2 O 5 (OH) 4 ) as well as quartz (SiO 2 ) ( Supplementary Fig. S2 ). The origin of this clay layer, unexpected in a wetland, is discussed below in the Discussion section. Fe concentrations (an average of 1.9±0.7% w/w) in the soil profile at spot A decrease from 0 to 30 cm ( Supplementary Fig. S5 ), consistent with the increasing dissolved Fe(II) concentration in the porewater in the same depth range ( Fig. 2 ). At spot B, the Fe situation is similar in the 0–30 cm range, but a spike in Fe concentration is visible at 30–40 cm ( Supplementary Fig. S4 ), corresponding to pyrite precipitation at this depth ( Supplementary Fig. S2 ). The soil U profile shows high U concentrations (2,400–4,400 p.p.m. for spot A and 1,000–14,000 p.p.m. for spot B) restricted to shallow depths (0–25 cm for spot A and 0–40 cm for spot B) comparing with low U concentrations (40–120 p.p.m.) beneath. Soil-associated rather than porewater-associated U represents >99% of U in the wetland. The high U zone corresponds to the abovementioned clay layer and immediately adjacent depths. Scanning electron microscopic (SEM) observation of the 15–20 cm soil sample at spot A showed a majority of layered mineral particles, corresponding to the clay minerals detected by XRD. No detectable U was associated with these clay particles. However, a minor phase identified repeatedly by SEM as exhibiting a distinctive morphology and chemical composition ( Fig. 5 ) was shown by HRTEM to be amorphous aggregates ( Fig. 6 ). This phase contains Fe, P, Al, Si, O and U ( Fig. 5 , Supplementary Table S2 ). Similar aggregates were also observed at other depths (10–15 cm and 20–25 cm) corresponding to the clay layer at spot A ( Supplementary Fig. S7 ). We conclude that this amorphous Al-P-Fe-Si phase binds U and controls U mobility in the soil. 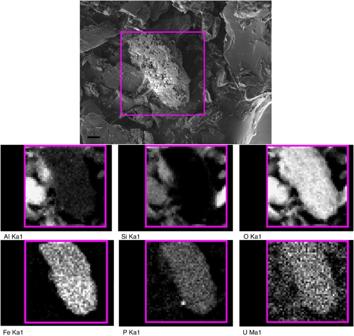Figure 5: SEM observation of U-containing aggregates in soil. SEM image and SEM-EDS mapping results of an aggregate exhibiting a morphology distinct from that of surrounding clay particles in the 15–20 cm soil sample at spot A. This aggregate contained Al and Si (albeit at lower concentrations than the surrounding aluminosilicates), O, Fe, P and U. Scale bar, 2 μm Figure 5: SEM observation of U-containing aggregates in soil. SEM image and SEM-EDS mapping results of an aggregate exhibiting a morphology distinct from that of surrounding clay particles in the 15–20 cm soil sample at spot A. This aggregate contained Al and Si (albeit at lower concentrations than the surrounding aluminosilicates), O, Fe, P and U. 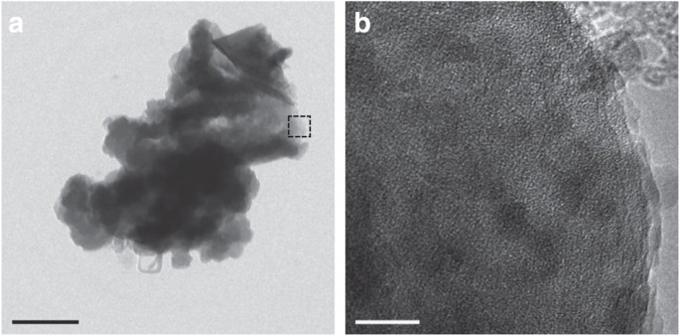Figure 6: TEM observation of U-containing aggregates in soil. (a) TEM and (b) HRTEM images of an U-containing amorphous aggregate in the 15–20 cm soil sample at spot A. The dashed square in the TEM image corresponds to the zone of HRTEM. Scale bar, 200 nm (a); 10 nm (b). Scale bar, 2 μm Full size image Figure 6: TEM observation of U-containing aggregates in soil. ( a ) TEM and ( b ) HRTEM images of an U-containing amorphous aggregate in the 15–20 cm soil sample at spot A. The dashed square in the TEM image corresponds to the zone of HRTEM. Scale bar, 200 nm ( a ); 10 nm ( b ). Full size image U redox and coordination was investigated by U L III -edge XAS on soil samples at 5–25 cm at spot A and at 5–40 cm at spot B, and the results are displayed in Fig. 7 . X-ray absorption near-edge structure (XANES) spectra exhibit an absorption maximum at 17,175.0 eV for all samples, underscoring the predominantly tetravalent oxidation state of U in the soil, which is consistent with the metal-reducing conditions evidenced by high Fe(II) concentrations in the porewater. Unfiltered and k 3 -weighted extended X-ray absorption fine structure (EXAFS) spectra collected for soil samples show oscillations similar to those of a monomeric U(IV) model compound, suggesting a similar atomic environment. Fits of EXAFS data further confirm the absence of a U–U pair correlation typical of U(IV) minerals and the presence of U(IV) coordinated to phosphate, a monomeric-U(IV)-like species. There is no evidence for U association with clays. Hence, we conclude that U in the soil is predominantly tetravalent and bound to the amorphous Al-P-Fe-Si aggregates through phosphate groups. 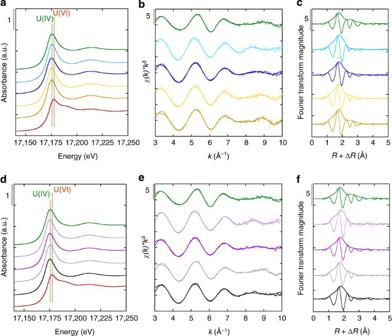Figure 7: XAS results from soil samples. Uranium LIII-edge data recorded for soil samples at 5–10 (light blue), 10–15 (deep blue), 15–20 (light yellow) and 20–25 cm (deep yellow) at spot A and those at 5–10 (light purple), 15–20 (deep purple), 20–25 (light grey) and 35–40 cm (black) at spot B compared with monomeric U(IV) (green) and U(VI)-acetate (red) model compounds. (a) XANES data of spot A showing that U(IV) is the predominant valence state in soil samples; (b) unfilteredk3-weighted EXAFS data of spot A; (c) magnitude and imaginary part of the Fourier transform (FT) of spot A; (d) XANES data of spot B showing that U(IV) predominates in the soil samples; (e) unfilteredk3-weighted EXAFS data of spot B; (f) magnitude and imaginary part of the FT of spot B. Experimental and calculated curves (seeSupplementary Table S3for fitting parameters) are displayed as solid and dashed lines, respectively. The vertical-dashed lines labelled ‘U(IV)’ and ‘U(VI)’ inaanddshow the energy of the U(IV) and U(VI) white lines, respectively. The vertical lines labelled ‘1’, ‘5’ and ‘5’ at the top left-hand corner ofaandd,bande,candfrepresent the scale ofyaxis. Figure 7: XAS results from soil samples. Uranium L III -edge data recorded for soil samples at 5–10 (light blue), 10–15 (deep blue), 15–20 (light yellow) and 20–25 cm (deep yellow) at spot A and those at 5–10 (light purple), 15–20 (deep purple), 20–25 (light grey) and 35–40 cm (black) at spot B compared with monomeric U(IV) (green) and U(VI)-acetate (red) model compounds. ( a ) XANES data of spot A showing that U(IV) is the predominant valence state in soil samples; ( b ) unfiltered k 3 -weighted EXAFS data of spot A; ( c ) magnitude and imaginary part of the Fourier transform (FT) of spot A; ( d ) XANES data of spot B showing that U(IV) predominates in the soil samples; ( e ) unfiltered k 3 -weighted EXAFS data of spot B; ( f ) magnitude and imaginary part of the FT of spot B. Experimental and calculated curves (see Supplementary Table S3 for fitting parameters) are displayed as solid and dashed lines, respectively. The vertical-dashed lines labelled ‘U(IV)’ and ‘U(VI)’ in a and d show the energy of the U(IV) and U(VI) white lines, respectively. The vertical lines labelled ‘1’, ‘5’ and ‘5’ at the top left-hand corner of a and d , b and e , c and f represent the scale of y axis. Full size image Analytical results show that the mineralogical composition of the U-bearing clay layer at spots A and B is similar to that of the clay deposit identified as overflow from the former settling pond ( Supplementary Figs S2 and S8 ), as is discussed in detail in Supplementary Note 1 . This strongly suggests that the clay layer within the wetland and the clay deposit in the overflow area share the same origin. The XAS results of the present field study evidence U(IV) binding to phosphate groups to form monomeric U(IV)-like species in the soil and are thus consistent with those of laboratory studies, which have previously demonstrated that U(VI) bioreduction could yield monomeric U(IV) characterized by U(IV) association to phosphate groups in batch and column systems [7] , [8] , [9] . In addition, abiotic U(VI) reduction via PO 4 3− -sorbed magnetite (Fe 3 O 4 ) and vivianite (Fe 3 (PO 4 ) 2 ) [11] also produced a similar product. Interestingly, in another site also located in the same Massif Central region, Fe-rich particulate Si gels were observed in the surface water under oxic conditions with U(VI) in association with these phases [17] , underscoring the complex chemistry of U. The high concentration of soluble U(IV) throughout the porewater profile while soil U(IV) is restricted to the top 30 cm is attributed to its mobility owing to its association with Fe(OH) 2 -OM colloids. The results in the present study demonstrate that U(IV) species in the porewater are distinct from those present in the soil in this wetland. This finding suggests that U(IV) bound to amorphous Al-P-Fe-Si aggregates in the soil is labile and complexes with mobile Fe and OM colloids. We propose that mobile OM-rich colloids form in the organic-rich layers and associate with Fe(II) originating from active Fe(III) reduction. The colloids are transported to the U-rich clay layer, where U(IV) may be transferred from the Al-P-Fe-Si aggregates in soil to the porewater colloids, because of the lability of the U-bearing soil aggregates. The presumed lability of this form of U(IV) is consistent with recent findings showing that monomeric U(IV), in contrast to UO 2 , appears to be mobile and reactive [18] . Moreover, the lability of U in a wetland soil reported by Schöner et al . [19] was attributed to the presence of amorphous U(VI) rather than U(IV) phases despite the prevalence of reducing conditions because it was not conceivable at the time that U(IV) could be present in a non-crystalline form. However, the present study reveals a more likely interpretation of those data with the formation of labile non-crystalline U(IV) species in the soil. Finally, as the composition of the stream colloids remarkably resembles to that of the U-bearing porewater colloids, it is conceivable that the release of U from the wetland is due to the migration of mobile porewater colloids into the stream water. A scheme summarizing the entire process is presented in Fig. 8 . 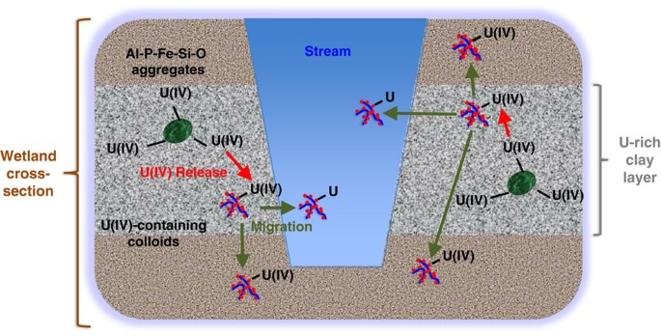Figure 8: Model of U release. The Fe- and OM-rich colloids are transported to the U-rich clay layer where some U(IV) is transferred from the Al-P-Fe-Si aggregates in soil to the porewater colloids, because this form of U(IV) is labile. Migration of mobile porewater colloids into the stream water then leads to the release of U from the wetland into the stream. Figure 8: Model of U release. The Fe- and OM-rich colloids are transported to the U-rich clay layer where some U(IV) is transferred from the Al-P-Fe-Si aggregates in soil to the porewater colloids, because this form of U(IV) is labile. Migration of mobile porewater colloids into the stream water then leads to the release of U from the wetland into the stream. Full size image U(IV) association to colloids in natural environments was suspected but never proven in numerous U solubility or mobility studies. For instance, Ollila et al . [20] , Noseck et al . [21] and Delecaut et al . [22] observed that the solubility of U under reducing conditions exceeded the solubility limit of the U(IV) phase. To explain their results, they speculated that U(IV) colloids enhanced the observed U(IV) solubility in experiments with groundwater from granitic bedrock, a uranium ore deposit or porewater from Boom Clay, respectively. While U(VI) mobility in association with colloids has been documented in the field [23] , [24] , [25] , and recent laboratory studies evidenced the formation of U(IV) silicate colloids ⩽ 20 nm in size [26] and that of U IV O 2 colloids [27] , this study is the first to demonstrate the association of U(IV) with colloids in natural environments and its resulting increased mobility. Reductive precipitation of uranium minerals is regarded as a major and sustainable mechanism to control U mobility. This mechanism is targeted by constructed wetland systems [6] that aim at stimulating microbial-mediated reduction of uranyl ions as described by Lovley et al . [13] Recent work has shown that the dominant species formed in the field by microbially mediated U(VI) reduction is monomeric U(IV) [10] . The present study further shows that the lability of non-crystalline U(IV) species may lead to the release of highly mobile U(IV)-bearing colloids. Both the formation of labile U(IV) and the potential release of U(IV)-bearing colloids should be considered carefully when designing wetland-based U remediation strategies. Stream water sampling and analysis The stream flowing through the wetland is shallow, with a maximum depth of ~20 cm. Stream water was sampled from a depth of ~10 cm. The sampling took place at various locations in April and November 2011 and July 2012, and each sample was divided into two parts, one of which was measured for pH (using WTW Multi 350i or HORIBA W20 multiparameter instruments) and alkalinity (using HACH titration cartridge with sulphuric acid and bromocresol green/methyl red colour indicators) and the other was filtered using 0.22 μm pore-size polyethersulfone (PES) membranes and analysed for U content using inductively coupled plasma mass spectrometry on a Thermo X7 analyser (detection limit for U: 4.2 nM). The pH and alkalinity values are reported in Supplementary Table S4 , and the U concentrations are shown in Fig. 1 . Stream water was also sampled near location 3 in Fig. 1 , filtered using 0.22 μm pore-size PES membranes and dried at 100 °C to obtain a powder. A part of the powder was dissolved completely using a three-step HNO 3 /HF microwave digestion procedure with a high-performance microwave and then analysed using inductively coupled plasma optical emission spectroscopy (ICP-OES) for main elements and U content, and another part was analysed using XRD for mineralogy. The results are shown in the main text and in Supplementary Fig. S2 . Porewater and soil sampling Soil and porewater sampling campaigns were carried out in November 2011 and July 2012. Soil core samples were only collected in November 2011, and porewater was sampled both in November and July to capture seasonal variations. The core was sampled under a high-flow Ar stream, sealed in airtight sterile bags and then conditioned in an anoxic chamber (N 2 atmosphere) 5 min away from the sampling spots. The vertical soil core was collected using a Russian corer, cut into 5 cm slices and each slice divided into two fractions, one of which was sealed in 0.127-mm-thick (0.005 inches) MYLAR bags and was stored at 4 °C for XAS analysis, and the other was dried by heating at 80 °C in an anoxic chamber for 24 h and then ground and homogenized to a fine powder for the remainder of the analyses. The porewater was sampled with a vertical resolution of 5 cm using multi-chambered piezometers designed and manufactured at EPFL. The concept of the piezometers is illustrated in Supplementary Fig. S9 . The piezometers were installed at spot A and spot B in April and June 2011, respectively, with the help of a peat soil corer [28] . The porewater in each chamber was pumped to the surface using a LAMBDA HIFLOW peristaltic pump and Tygon R-3603 tubing, and the pH and DO of the porewater was measured using airtight flow-through cells custom made for the probes at EPFL. The porewater was then sampled under a high-flow Ar stream, sealed in serum bottles with blue butyl rubber stoppers and then handled in an anoxic chamber (N 2 atmosphere) 5 min away from the sampling spots. In the anoxic chamber, the samples were filtered using 0.22 μm pore-size PES membranes, and divided into three fractions: one amended with anoxic 2 M HCl (1:1 volume ratio) for Fe(II) analysis, one amended with 5 M HNO 3 (1:5 volume ratio) for metal ion analysis and the rest stored in a serum bottle sealed with a butyl rubber stopper for the remainder of the analyses. Analysis of porewater chemistry The Fe(II) concentration in porewater samples was determined using the ferrozine colorimetric method described by Stookey [29] . A solution of ferrozine [3-(2-pyridyl)-5,6-bis(4-phenylsulfonic acid)-1,2,4-triazine] was prepared at 1 g l −1 in 50 mM HEPES at pH 7.0. Acidified porewater samples were analysed by mixing 15 μl of sample with 1,485 μl of ferrozine solution. The absorbance at 562 nm was measured with a Shimadzu UV-2501 PC spectrophotometer. Metal ion concentrations in porewater samples were obtained using ICP-OES on a Shimadzu ICPE-9000 analyser (respective detection limit for Fe and U: 1.8 and 21 nM). Anion concentrations were measured using a Dionex ICS 3000 ion chromatograph. Dissolved organic carbon and dissolved inorganic carbon (bicarbonate) in porewater were analysed using a Shimadzu TOC-Analyzer 5000 (detection limit: 16.7 μM). Laser-induced fluorescence spectroscopy The samples for LFS analysis were prepared at EPFL in an H 2 /N 2 (3–4% H 2 ) anoxic chamber. Two spot A porewater samples from November (15–20 and 35–40 cm) and one from July (15–20 cm) were selected for LFS analysis. LFS is only able to detect dissolved U(VI). Each sample was divided into two 4 ml subsamples acidified using 1 ml of N 2 -purged anoxic 1 M HCl to release U from the Fe-rich colloids. Previous tests showed that no U(VI) could be detected if it was bound to Fe-rich colloids. One subsample was sealed in a serum bottle with a butyl rubber stopper until the analysis, and the other was exposed to air for at least 24 h to oxidize U(IV) to U(VI). The samples were then sent to HZDR for analysis. On arrival, the serum bottles containing anoxic subsamples were opened in a glove box (Braun, Germany) with an N 2 atmosphere (<6 p.p.m. O 2 ), and the oxidized ones were opened to the air. The subsamples were transferred into a plastic cuvette and sealed with a teflon plug. The closed cuvette was then stored for 24 h in a freezer at 253 K. The formed ice block was extracted from the cuvette and immediately transferred to the cold gas system sample holder. This cold gas system allows cooling the sample to 120 K by use of N 2 gas from a liquid nitrogen source (Isotherm, Germany). Acquiring spectra at this temperature minimizes the quenching effect of chloride in the samples. The thermostat housing has three windows, where two opposing windows allow the laser beam through while the third, at a right angle, is used for collecting the emitted luminescence. The luminescence light is focused onto an optical fibre and transmitted into a spectrograph (Acton Research, USA). The resolved spectrum is measured by an intensified charge-coupled device camera system (Roper Scientific, USA). A laser source (Inlite, Continuum, USA) is used for U excitation. The fourth harmonic of a Nd:YAG laser (wavelength=266 nm) was used to excite the uranium(VI) species in the frozen sample. The duration of the laser pulses was 10 ns. The repetition rate of the laser was 20 Hz and the energy of the laser pulses was adjusted to about 5 mJ. The measurement by the camera system started immediately after application of the laser pulse (30 ns). The gate width of the camera was set to 500 μs. Three hundred laser shots were collected for each spectrum and repeated three times. Because of the low luminescence intensities detected, no time-resolved spectra were collected. Ultrafiltration Ultrafiltration of the porewater samples was performed in July 2012. The system consisted of a 0.45-μm pre-filtration through a cellulose acetate in-line filter, followed by parallel filtration through a 0.22-μm pore-size Millipore PES membrane and ultrafiltration through 500 and 10 kDa pore-size Millipore Biomax PES membranes. These membranes were secured in stainless steel mounts, with polytetrafluoroethylene (PTFE)-coated inner walls to prevent metal contamination. The whole procedure was performed in an anoxic glove bag purged and filled with N 2 gas. Blank samples were obtained for each filtration threshold by running ultrapure water through the system. Between each sample, the cleaning procedure consisted of rinsing the entire system with 2% HNO 3 followed by ultrapure water until the pH was back to neutral. Electron microscopy SEM observation on selected soil samples was conducted without C coating using a Carl Zeiss Merlin microscope with GEMINI II column at 1 kV and 100 pA at EPFL. TEM observation was conducted on selected porewater and soil samples at EPFL. The TEM grids and windows were prepared in an H 2 /N 2 (3–4% H 2 ) anoxic chamber. For the porewater sample, several microlitres were extracted by a needle and a syringe and dropped onto the TEM SiN window. The liquid was left on the window for about 10 s and then wicked away using a paper towel. This procedure was repeated three to five times. TEM observation showed that porewater colloids were loaded onto the grid. For soil samples, finely ground dry soil powder was loaded onto C-coated TEM grids by spraying powder onto the grid. The grids and the windows were transferred to the microscope in an anoxic jar. The chemical composition of porewater colloids and soil U-rich aggregates was studied by scanning TEM and X-ray energy-dispersive spectroscopy (EDS) in an FEI Tecnai Osiris microscope at 200 kV (FEI, Eindhoven, The Netherlands) equipped with four windowless Super-X silicon drift detector (SDD) EDX detectors. Quantitative EDS results were obtained with Bruker Esprit software (Bruker Corporation). The morphology and phase composition were studied by conventional and HRTEM (TEM and HRTEM) and electron diffraction in an FEI CM300UT/FEG microscope at 300 kV (FEI). Images and SAED patterns were recorded on a Gatan 797 slow scan charge-coupled device camera and processed with the Gatan Digital Micrograph software (Gatan, Inc., Pleasanton, CA, USA). Phase identification was performed by analysing SAED patterns using a software known as JEMS ( http://www.cimewww.epfl.ch/people/stadelmann/jemsWebSite/jems.html ) for the electron-optical parameters of the microscope and the structural data of Fe oxides (27856) and hydroxides (53992) taken from the Inorganic Crystal Structure Database, FIZ Karlsruhe, Germany and NIST, US Department of Commerce, 2013. Analysis of soil chemistry Water content of the soil samples was obtained by weighing the samples before and after drying. Soil TOC content was measured in dried homogenized samples with a Shimadzu TOC-V CPH/CPN analyser. To study the soil chemical composition and U content, soil samples were dissolved completely using a three-step microwave digestion procedure with a high-performance microwave (Microwave Laboratory Systems). Hundred milligrams of dried and homogenized sample was mixed first with 4 ml of HNO 3 (65%) and 4 ml of H 2 O 2 , and the first microwave digestion step (all steps were carried out at 100 °C) was started followed by the second, which involved the addition of 2 ml of HF (48%), and finally the third with the addition of 20 ml of H 3 BO 3 (4.5%). The final extract was diluted with MilliQ water to 100 ml and analysed using ICP-OES for main elements and U content. The main elements’ composition is shown in Supplementary Fig. S5 . X-ray diffraction To avoid oxidation by air during analysis, XRD analysis was conducted under anoxic conditions at the Institut de Minéralogie et de Physique de Milieux Condensés (IMPMC) in Paris. Finely ground dry soil samples were sealed in serum bottles with butyl rubber stoppers before analysis. Powder samples were loaded onto a Si single crystal ‘zero diffraction plate’ under a N 2 atmosphere in a Jacomex glove box (O 2 ⩽ 20 p.p.m.) at IMPMC. XRD measurements were performed with Co Ka (6.93 keV, wavelength=1.79 Å) radiation on a Panalytical X’Pert Pro MPD diffractometer mounted in Debye–Scherrer configuration using an X'Celerator detector to collect the diffracted beam. Data were recorded in the continuous-scan mode in the 3–80° 2 θ range with a step of 0.0330°. X-ray absorption spectroscopy The monomeric U(IV) model compound was obtained by following the procedure described by Bernier-Latmani et al ., [7] whereas the U(VI)-acetate model compound was prepared by diluting U(VI)-acetate powder (Fluka) into cellulose. Soil samples for XAS analysis were mounted onto sample holders, sealed in individual MYLAR bags (0.127 mm thick) and sealed in a metallic jar at EPFL in an H 2 /N 2 (3–4% H 2 ) anoxic chamber. The jar was then shipped to XAS beamlines and was kept sealed until analysis. Uranium L III -edge (17.166 keV) XANES and EXAFS data of selected spot A and spot B samples were obtained at the Core EXAFS beamline (B18) of Diamond Light Source and Rossendorf Beamline (BM20) of the European Synchrotron Radiation Facility, respectively. On analysis, the sample was mounted quickly onto the cryostat rod and inserted into the cryostat. XANES data showed no evidence of air-induced oxidation with this approach. We collected XANES and EXAFS data in fluorescence mode under N 2 -liquid temperature (~77 K) at B18 of Diamond Light Source or He-liquid temperature (~10 K) at BM20 of European Synchrotron Radiation Facility. The Si(111) double-crystal monochromator was used in channel-cut mode. The spectra were collected in fluorescence mode using multielement solid-state Ge detector, together with I 0 , I 1 and I 2 signals using ionization chambers. Energy was calibrated by using double-transmission set-up in which a uranium L III -edge spectrum of the sample and that of Y metal (first inflection point at 17,038 eV) foil reference sample placed between I 1 and I 2 were simultaneously recorded. Several EXAFS scans were summed for each sample to obtain an adequate signal-to-noise ratio at k =10 Å −1 . Athena of IFEFFIT program package [30] was used for normalization and background removal. The EXAFS oscillations were extracted from raw spectra by standard methods including a spline approximation for the atomic background. Artemis of IFEFFIT program package was used for shell-by-shell fitting of EXAFS data. Theoretical backscattering phase and amplitude functions were calculated with the FEFF 8.4 code [31] using Artemis. The Fourier transform peaks are shifted to lower values, R +Δ R , relative to the true near-neighbor distances, R , due to the phase shift of the electron wave in the adjacent atomic potentials. This Δ R shift is considered as a variable during the shell fits. The data-fitting ranges were k =3–11 Å −1 and R +Δ R =1–3.5 Å for the EXAFS and Fourier back transform, respectively. The amplitude reduction factor, S 0 2 , was defined as 0.9 in the data fits. Numerical constraints were applied to keep the values of the fits within a physically reasonable range, and the number of free parameters was kept maximally at four for most cases. How to cite this article: Wang, Y. et al . Mobile uranium(IV)-bearing colloids in a mining-impacted wetland. Nat. Commun. 4:2942 doi: 10.1038/ncomms3942 (2013).